Energy and angular momentum balance in wall-bounded quantum turbulence at very low temperatures A superfluid in the absence of a viscous normal component should be the best realization of an ideal inviscid Euler fluid. As expressed by d’Alembert’s famous paradox, an ideal fluid does not drag on bodies past which it flows, or in other words it does not exchange momentum with them. In addition, the flow of an ideal fluid does not dissipate kinetic energy. Here we study experimentally whether these properties apply to the flow of superfluid 3 He-B in a rotating cylinder at low temperatures. It is found that ideal behaviour is broken by quantum turbulence, which leads to substantial energy dissipation, as was also observed earlier. Remarkably, the angular momentum exchange between the superfluid and its container approaches nearly ideal behaviour, as the drag almost disappears in the zero-temperature limit. Here the mismatch between energy and angular momentum transfer results in a new physical situation, with severe implications on the flow dynamics. A remarkable property of incompressible and inviscid potential flow, as discovered by d’Alembert in the mid eighteenth century, is that bodies moving at a constant velocity relative to this ideal fluid experience no drag [1] . This gross contradiction with observations of real fluids was resolved in the beginning of the twentieth century by Prandtl who introduced the concept of a boundary layer obeying the no-slip boundary condition. Rapid spatial variation of the velocity in the boundary layer sustains viscous effects that lead to drag at all Reynolds numbers. In superfluids, at temperatures much below the critical temperature T c , the viscous normal component is almost absent. The superfluid component might seem to be close to an ideal fluid considered by d’Alembert, both in the bulk, where vortex-free flow is potential, and at the boundaries, where the no-slip condition of viscous fluids reduces to the ‘no flow through the boundary’ condition. In reality, however, the dynamics of different non-trivial superfluid flows also include the motion of quantized vortex lines. In many cases, this takes the form of quantum turbulence, that is, the complex motion of tangled and reconnecting vortices. It has been demonstrated recently that quantum turbulence breaks the correspondence between superfluids and ideal fluids. In particular, finite energy dissipation and, thus, finite effective viscosity or friction have been observed in low-temperature helium superfluids [2] , [3] , [4] , [5] , and were in some cases linked to a quasiclassical turbulent energy cascade [5] , [6] . However, an intriguing question is whether low-temperature quantum turbulence also mimics viscous boundary flow by producing similar drag. So far, measurements of the superfluid drag in the T →0 limit have been performed only for flows around various oscillating objects [7] , [8] , [9] . In these experiments, the ideal boundary conditions have not been necessarily satisfied, owing to surface pinning, and substantial drag was measured, approaching in magnitude to that of the normal fluid [9] . Our measurement of energy dissipation and momentum exchange with the container walls in steady-state turbulent flow is outlined in Fig. 1 . We measured the motion of a turbulent vortex front propagating along a rotating cylinder filled with superfluid 3 He in the B-phase. We used a container with very smooth walls, which means that practically pinning was excluded and ideal flow boundary conditions were restored. This is possible in 3 He-B because of the large vortex core radius ( a ~0.1 μm at 0.5 bar liquid pressure). 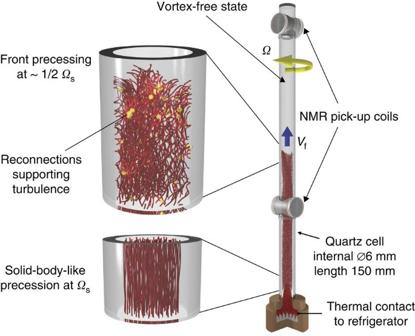Figure 1: Turbulent vortex front motion in a rotating cylinder. The front moves axially upward and rotates azimuthally with respect to the cylinder. The motion is detected with two NMR pick-up coils, which are 9 cm apart. In the front, where the vortices bend perpendicular to the side wall, the angular velocity of the superfluid and also the precession frequency of the vortices changes from zero toΩsΩ. The difference in the average precession frequencies between the front and the vortex bundle behind it enforces reconnections (yellow dots) and turbulence in the front, as seen in the zoomed view on the top left. The differential precessions also wind the vortex lines behind the front to a twisted configuration21. This snapshot of the ensuing vortex configuration comes from numerical calculations at 0.27Tc. Figure 1: Turbulent vortex front motion in a rotating cylinder. The front moves axially upward and rotates azimuthally with respect to the cylinder. The motion is detected with two NMR pick-up coils, which are 9 cm apart. In the front, where the vortices bend perpendicular to the side wall, the angular velocity of the superfluid and also the precession frequency of the vortices changes from zero to Ω s Ω . The difference in the average precession frequencies between the front and the vortex bundle behind it enforces reconnections (yellow dots) and turbulence in the front, as seen in the zoomed view on the top left. The differential precessions also wind the vortex lines behind the front to a twisted configuration [21] . This snapshot of the ensuing vortex configuration comes from numerical calculations at 0.27 T c . Full size image As a result, we find that a boundary layer similar to that in classical fluids was not created. In the front motion, exchange of momentum with the walls turned out to be significantly suppressed in comparison with energy dissipation. This discrepancy between the nearly ideal liquid behaviour with respect to drag and the more enhanced dissipative behaviour with respect to energy transfer changes the T →0 dynamics of quantum fluids in a profound manner. In this regime, the proper description of wall-bounded quantum turbulence requires two effective friction parameters, one for energy dissipation and another for momentum coupling, which become substantially different at the lowest temperatures. In particular, as the amount of the transferred momentum is reduced, the superfluid starts to decouple from the moving solid surface. Here the slow laminar dynamics allow for more balanced momentum exchange with the walls via the diluted normal component and, thus, the role of laminar flow becomes substantially enhanced compared with what one would expect from higher temperatures. Axial velocity of vortex front The measurement starts with the container at rest, with vortex-free non-rotating superfluid. When the container is set into rotation at an angular velocity Ω , a turbulent front forms at the rough surfaces of the heat exchanger at the bottom and starts to move upwards along the cylinder, bringing the superfluid behind it into rotation [4] . The axial front velocity V f is determined from the flight time between two pick-up coils of NMR spectrometers. The energy dissipation rate can be inferred from V f by considering the free-energy difference of the superfluid before and after the front. The validity of this approach was proven by direct calorimetric measurement of the dissipated heat in the front propagation [10] . The rate of the angular momentum exchange with the bounding walls can be determined either directly from the rotation Ω s of the superfluid behind the front or indirectly from the dependence of V f on Ω . We first discuss the indirect approach. The measured axial front velocity is presented in Fig. 2 as a function of Ω at constant temperature and as a function of temperature at constant Ω . As seen from Fig. 2a , the Ω dependence of V f gradually changes from linear V f Ω towards quadratic V f Ω 2 , with decreasing temperature below 0.3 T c . From Fig. 2b , one finds the limiting behaviour as a function of temperature; at high temperatures, the normalized front velocity approaches the Ω -independent ‘single-vortex-result’ [4] V f /( ΩR )≈ α ( T ), and below 0.2 T c it appears to level off to a T -independent but Ω -dependent value. Here R is the radius of the cylinder and α ( T ) is the dissipative mutual friction parameter, which characterizes the coupling of the normal and superfluid components of 3 He-B via scattering of the thermal quasiparticle excitations from the vortex cores [11] . At the lowest temperatures, the interquasiparticle collisions are absent, the excitations move along ballistic flight paths and the friction is exponentially reduced as α exp(−Δ/ T ), where Δ is the superfluid energy gap. 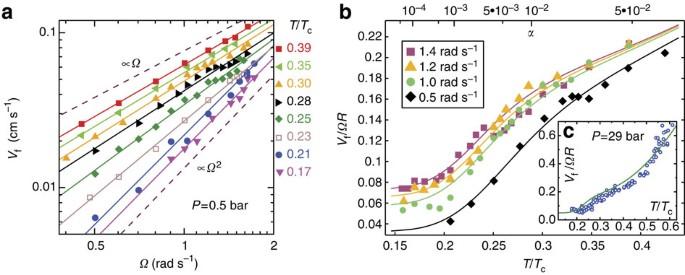Figure 2: Axial front velocity and fits to the model equation (2). (a) VelocityVf(T,Ω) plotted versus the angular velocity of rotationΩ, with logarithmic axes. The dashed lines correspond toVfΩandVfΩ2for comparison. (b) Dependence ofVf/(ΩR) on temperatureTat four differentΩ. In theT→0 limit,Vftends to aT-independent butΩ-dependent value determined by the residual termsand. On the top horizontal axis, the mutual frictionα(T) is given13. (c) In the inset, the data onVf(T) measured at 29 bar pressure in ref.4forΩ≈1 rad s−1is compared with equation (2), using the measuredα(T) for 29 bar22and the same values for the four fitting parameters as obtained from the present 0.5 bar measurements. Figure 2: Axial front velocity and fits to the model equation (2). ( a ) Velocity V f ( T , Ω ) plotted versus the angular velocity of rotation Ω , with logarithmic axes. The dashed lines correspond to V f Ω and V f Ω 2 for comparison. ( b ) Dependence of V f /( ΩR ) on temperature T at four different Ω . In the T →0 limit, V f tends to a T -independent but Ω -dependent value determined by the residual terms and . On the top horizontal axis, the mutual friction α ( T ) is given [13] . ( c ) In the inset, the data on V f ( T ) measured at 29 bar pressure in ref. 4 for Ω ≈1 rad s −1 is compared with equation (2), using the measured α ( T ) for 29 bar [22] and the same values for the four fitting parameters as obtained from the present 0.5 bar measurements. Full size image Phenomenological model of front propagation The front propagation can be understood using a phenomenological model based on the consideration of energy and angular momentum balance in the front. The model relies on the equation of superfluid hydrodynamics averaged over vortex lines [12] , which is basically the Euler equation with an additional friction force from the normal component and a line-tension force owing to the quantum nature of vortices. The friction force is parametrized with α ( T ), whereas the tension-force parameter is λ =( κ /4π)ln( l / a ), where κ = h /(2 m 3 )≈0.07 mm s −2 is the quantum of circulation and l ≈(2 Ω s / κ ) −1/2 ≈0.1 mm is the inter-vortex distance. Strictly speaking, these equations are applicable only when the vortex lines are locally roughly parallel to each other. To allow an extension to the case of the turbulent front, we replace the friction α with two separate effective friction parameters: α en when we consider the energy balance and α am for the angular momentum balance. These parameters are defined as follows: Here C en , C am ≈1 account for the modification of the friction from the normal component owing to the reduced polarization of the vortex lines and their fluctuating motion in the turbulent front. The parameters and describe the contribution of turbulence and possible effects from residual surface friction. For simplicity, we consider all four phenomenological parameters to be ( T , Ω ) independent. Analysis of the energy and the angular momentum balance (see the Supplementary Discussion for details) leads to the following expressions for the front velocity V f and the angular velocity Ω s of the superfluid behind the front: The expression for V f is a direct generalization of the laminar single-vortex result. The expression for Ω s follows from balancing the azimuthal components of the friction and line-tension forces. The friction force appears because the azimuthal velocities of the normal and superfluid components differ, whereas the line-tension force is due to the twisting of the vortices behind the front. The expression for the front velocity V f (equation 2) is compared in Fig. 2a with its measured values in the temperature range, where the mutual friction α ( T ) changes by roughly three orders of magnitude. The solid lines show the model (2) with the four fitting parameters C en =0.52, C am =1.33, and . The temperature dependence α ( T ) is taken from the measurements in ref. 13 . The model seems to be in good agreement with the measurements and, in particular, reproduces all the qualitative features of V f ( T , Ω ) discussed above. Direct measurement of superfluid angular velocity Occasional small axial asymmetries in the precessing front and in the bundle behind it cause oscillations in the NMR signal [10] . In such cases, the superfluid angular velocity Ω s can be directly extracted from the frequency of the oscillations, albeit usually in a limited range of temperatures slightly above 0.2 T c . This allows us to determine the angular momentum coupling parameter α am = λΩ s /( R 2 Ω ( Ω − Ω s )) independently of the front velocity V f . The results shown in Fig. 3 highlight again the good agreement with the fitted parameter values extracted from Fig. 2 and the two orders of magnitude difference between α en = V f / Ω s R and α am . 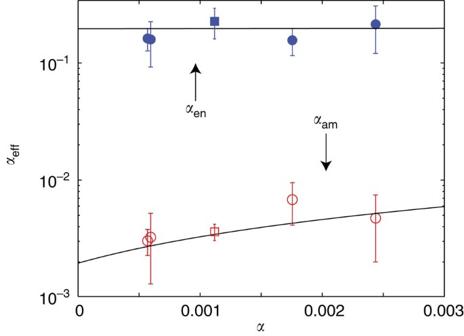Figure 3: Direct measurement of the effective friction parameters and comparison with the model. The data pointsαamandαenhave been extracted from direct simultaneous measurements of azimuthal precessionΩs(T,Ω,P) and axial front propagation velocityVf(T,Ω,P) using equation (2), and are plotted as the function of temperature in terms of the measured mutual frictionα(T,P). The superfluid angular velocityΩsis measured from the precession frequency of the vortex bundle behind the front, withΩin the range 0.4–1.0 rad s−1using the method described in ref.10. Circles denote measurements atP=0.5 bar and squares at 29 bar. The solid lines represent equation (1) with the same parameters used to fit the velocity data inFig. 2. Figure 3: Direct measurement of the effective friction parameters and comparison with the model. The data points α am and α en have been extracted from direct simultaneous measurements of azimuthal precession Ω s ( T ,Ω, P ) and axial front propagation velocity V f ( T , Ω , P ) using equation (2), and are plotted as the function of temperature in terms of the measured mutual friction α ( T , P ). The superfluid angular velocity Ω s is measured from the precession frequency of the vortex bundle behind the front, with Ω in the range 0.4–1.0 rad s −1 using the method described in ref. 10 . Circles denote measurements at P =0.5 bar and squares at 29 bar. The solid lines represent equation (1) with the same parameters used to fit the velocity data in Fig. 2 . Full size image This difference and, in particular, the minute value of emphasize our central result. When the influence of the normal component on the energy dissipation and coupling to the container walls is excluded, α →0, the residual effective friction parameters and should be primarily associated with quantum turbulence in the front. The relatively large value of shows that turbulence in the front efficiently enhances energy dissipation. For comparison, the same friction from the normal component, α ≈0.2, is reached at T ≳ 0.45 T c , where the density of the normal component is about 30% of the total liquid density. The contribution of quantum turbulence to the dissipation in the zero-temperature limit is usually attributed to the energy transfer in the turbulent cascade to length scales much smaller than the inter-vortex distance, where it is dissipated by the emission of non-thermal quasiparticles from the vortex cores [14] . The much smaller residual term attests that the angular momentum transfer from the boundaries is much less effective, and that the drag from the superfluid on the boundaries almost disappears in the zero-temperature limit. It is not clear whether the value of should be completely ascribed to the residual friction in the motion of the surface-attached vortices or whether it has a contribution from turbulence, such as momentum transfer from cascading effects, similar to those in the energy dissipation or via annihilation of small vortex loops at the surfaces. There are some arguments in favour of the turbulent contribution. First, the value of is four times larger than the residual friction term in laminar vortex motion [13] . In addition, Figs 2c and 3 demonstrate that the same fitted effective friction parameters explain earlier high-pressure measurements [4] , which were conducted in a different quartz cylinder. We take this to indicate that the model parameters are not strongly dependent on our surfaces or on the pressure-dependent vortex core radius. To summarize, we find that two separate effective friction parameters have to be introduced to account for energy and angular momentum transfer, respectively. By comparing the measurements with a phenomenological model of turbulent front propagation, it is seen that these parameters differ by two orders of magnitude. This difference leads to new physical effects in superfluid dynamics in the T →0 limit, such as the recently observed decoupling from the reference frame of the container [10] . Decoupling of the superfluid and normal components is also discussed, for instance, in the evolution of a rotating neutron star [15] when it cools through T c , but here in the T →0 limit the mechanism of decoupling is different. It leads to the unusual situation that efficient energy dissipation is achieved in turbulent bulk flow, but the angular momentum exchange is not enhanced as much beyond that provided by the bulk mutual friction coupling; thus, a turbulent boundary layer, similar to that in the classical case, is not formed. Sample preparation and triggering vortex motion The measuring setup consists of a long cylinder made from fused quartz and filled with liquid 3 He-B at 0.5 bar pressure. The internal surfaces of the cylinder are treated with hydrofluoric acid [16] and are appropriately cleaned to remove pinning sites for vortices. At its bottom end, the cylinder opens to a sintered-silver heat exchanger. Its rough surface ensures that vortices are formed there at low rotation velocity. In the experiment, we rapidly increase the rotation velocity from zero to the desired target velocity Ω . This creates a turbulent burst at the bottom end and triggers an upward-propagating vortex front. Owing to the smooth walls, the critical velocity of vortex formation is as high as 1.8 rad s −1 elsewhere in the quartz cylinder, and at lower velocities than this volume above the front remains in the meta-stable vortex-free Landau state, which eventually is displaced by the front. The final state, which is reached only long after the front has reached the end of the cylinder via laminar spin-up of vortices [17] , is the equilibrium vortex state with a constant solid body density of rectilinear line vortices. After each measurement, rotation is stopped and the sample is warmed up to ~0.7 T c for about 1 h, to allow remanent vortices to annihilate [18] before cooling down again for a new measurement. Alternatively, the sample may be warmed up above the T c on which it can be cooled down immediately. NMR detection techniques and thermometry The propagation of the front is monitored with two NMR pick-up coils. At temperatures above 0.2 T c and velocities above 0.6 rad s −1 , the arrival of the front can be detected by tracing the NMR signal at the so-called counterflow peak in the linear NMR spectrum [19] . The arrival is seen as a rapid decrease of the NMR absorption. This method loses sensitivity at lower rotation velocities and temperatures, as the counterflow peak rapidly decreases in amplitude. There the front propagation is monitored from the frequency of the coherent non-linear NMR signal generated by a Bose–Einstein condensate of magnon quasiparticles in a magnetic trap in the middle of the pick-up coil. This frequency depends strongly on the difference in the velocities of the azimuthal flow of the normal and the superfluid components, which provides a contribution to the radial trapping of the magnon condensate [20] . A small axial pinch coil is used around the NMR pick-up coil to provide the localization of the trap in the axial direction. The temperature is determined from the resonance width of a quartz tuning fork oscillator, located close to the heat exchanger, which depends on temperature as in the ballistic regime of quasiparticle transport. How to cite this article: Hosio, J.J. et al . Energy and angular momentum balance in wall-bounded quantum turbulence at very low temperatures. Nat. Commun. 4:1614 doi: 10.1038/ncomms2618 (2013).